Selenoether oxytocin analogues have analgesic properties in a mouse model of chronic abdominal pain Poor oral availability and susceptibility to reduction and protease degradation is a major hurdle in peptide drug development. However, drugable receptors in the gut present an attractive niche for peptide therapeutics. Here we demonstrate, in a mouse model of chronic abdominal pain, that oxytocin receptors are significantly upregulated in nociceptors innervating the colon. Correspondingly, we develop chemical strategies to engineer non-reducible and therefore more stable oxytocin analogues. Chemoselective selenide macrocyclization yields stabilized analogues equipotent to native oxytocin. Ultra-high-field nuclear magnetic resonance structural analysis of native oxytocin and the seleno-oxytocin derivatives reveals that oxytocin has a pre-organized structure in solution, in marked contrast to earlier X-ray crystallography studies. Finally, we show that these seleno-oxytocin analogues potently inhibit colonic nociceptors both in vitro and in vivo in mice with chronic visceral hypersensitivity. Our findings have potentially important implications for clinical use of oxytocin analogues and disulphide-rich peptides in general. Since its discovery over a century ago, few bioactive peptides have proven to be more important and widely studied than the peptide hormone oxytocin (OT) [1] . OT was the first peptide hormone to be sequenced and synthesized, an achievement recognized with the award of the 1955 Nobel Prize in Chemistry to Vincent du Vigneaud [2] . OT has since become widely used in obstetrics to induce labour, prevent post-partum haemorrhage and stimulate lactation in nursing mothers [3] . In the central nervous system, OT functions as a neurotransmitter involved in complex social interactions, including maternal behaviour, partnership and social bonding [4] . Recent studies have shown that OT function (and that of the closely related hormone vasopressin) is impaired in brain disorders associated with social dysfunction such as autism, social anxiety, stress and schizophrenia, triggering an explosion of interest in the use of OT for treatment of mental conditions [5] , [6] . OT receptors have also attracted attention for their role in memory [7] , breast cancer tumour growth [8] and visceral pain [9] , [10] . Nasal administration of OT reduces abdominal pain and discomfort in patients with chronic idiopathic constipation [9] , whereas continuous intravenous OT significantly increases thresholds for visceral perception in patients with Irritable Bowel Syndrome (IBS) [10] . The mechanisms underlying these effects remain unclear and are important to determine as chronic abdominal pain represents a major clinical problem, with IBS alone affecting ~11% of the Western population [11] . With many clinical trials currently underway to investigate OT effects in a wide range of diseases [12] it is imperative to advance strategies that improve the metabolic stability and drug-like properties of this unique signaling hormone and neurotransmitter. In this study, we disclose several insights into OT. We describe the well-defined structure of OT in aqueous solution and present an efficient strategy for production of more stable analogues based on seleno-chemistry. Finally, we demonstrate that OT receptor expression and function is significantly upregulated in colonic neurons of mice with chronic visceral hypersensitivity (CVH) and show that stable OT analogues are potently analgesic in this animal model of chronic abdominal pain. Taken together, our results indicate that stable OT analogues have significant potential for the treatment of chronic abdominal pain associated with conditions such as IBS. OT analogues with an engineered selenoether bridge OT is a cyclic peptide comprising nine amino-acid residues with a single disulphide bridge between the first and sixth residues. The disulphide bond is critical for binding to the OT receptor; however, it renders the peptide susceptible to endogenous reductive degradation [3] . Although replacement of the labile bridge with a more redox-stable linkage is an attractive approach to improve the metabolic integrity of OT, it is non-trivial for OT, as its biological activity is sensitive to minute structural modifications within the cyclic framework. Even minor distortions such as increasing the 20-membered ring by one methylene group [13] , substitution of Cys1 by penicillamine [14] or replacement of the disulphide bond by an amide [15] , lanthionine [16] or dicarba [17] bond leads to a significant decrease in agonist activity. In contrast, OT bioactivity is retained when the OT S-S bond is replaced by chalcogen linkages such as cystathionine (CH 2 -S, Ctt), diselenide (Se-Se), selenylsulphide (Se-S) and ditelluride (Te-Te) bonds, where the 20-membered ring framework is conserved [16] . Of particular interest for drug development is the close isomorphism between disulphides and non-reducible Ctt bonds [18] , [19] . Carbetocin, a Ctt analogue of desamino-OT, is an example of a long-acting disulphide bond mimetic that is approved as a drug [20] . Conventional intramolecular S -alkylation of cysteine used to build Ctt bridges in cyclic peptides is often problematic ( Fig. 1a ) and, with few exceptions [18] , [19] , [21] , [22] , has not found broad application in the field of peptide chemistry. Here we describe a macrocyclization strategy that exploits the advantageous physicochemical properties of selenocysteine (Sec, U) instead of cysteine to accomplish effective crosslinking that can be applied not only to native OT but also to a wide range of other peptide sequences. In recent years, Sec has been incorporated into several bioactive peptides with innovative properties [23] , [24] . For example, substitution of S-S bonds by isosteric Se-Se bonds can improve peptide folding and stability [25] , [26] , [27] . We envisaged that replacement of a disulphide bond (S-S, bond length 2.03 Å) [28] by a non-reducible selenocystathionine (SeCtt) bond (Se-C, bond length 1.95–1.99 Å) [28] might enhance the metabolic stability of cyclic peptides with minimal structural perturbation. Furthermore, the low p K a of the selenol in Sec [29] should allow selenide ring closure 1 to proceed efficiently under acidic to neutral conditions, largely preventing deterioration of labile electrophilic moieties at higher pH ( Fig. 1b ). 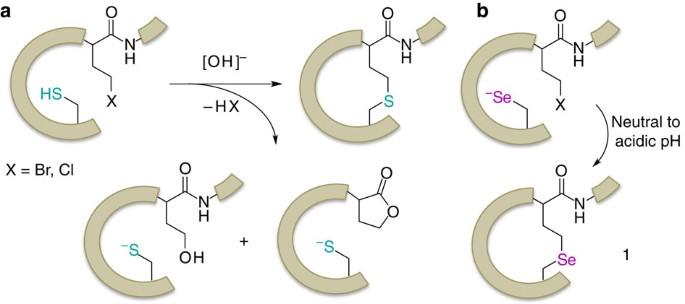Figure 1: Synthesis of Ctt and SeCtt cyclic peptides. (a) Synthesis of Ctt cyclic peptides by intramolecular SN2-substitution of a γ-halo-homoalanine by cysteine21,22and possible degradation products of the linear precursor. Under the basic conditions required for monosulphide cyclization, the γ-halo-homoalanine residue can undergo intramolecular lactonization or be hydrolyzed to homoserine. (b) Intramolecular ring closure of a SeCtt cyclic peptide. Figure 1: Synthesis of Ctt and SeCtt cyclic peptides. ( a ) Synthesis of Ctt cyclic peptides by intramolecular S N 2-substitution of a γ-halo-homoalanine by cysteine [21] , [22] and possible degradation products of the linear precursor. Under the basic conditions required for monosulphide cyclization, the γ-halo-homoalanine residue can undergo intramolecular lactonization or be hydrolyzed to homoserine. ( b ) Intramolecular ring closure of a SeCtt cyclic peptide. Full size image Synthesis of linear peptide precursors In order to investigate the scope of SeCtt cyclization in comparison with Ctt cyclization, a series of linear OT sequences featuring Sec, Cys and halogenated residues at the corresponding sites of the native Cys1–Cys6 disulphide bond were synthesized by solid-phase peptide synthesis (SPPS) ( Fig. 2 ). The linear precursors 2 , 3 and 4 were assembled on a Rink amide resin using standard Fmoc chemistry ( Fig. 2a ) [30] . The crucial chlorination step, where the tert- butyl dimethylsilyl (TBDMS)-protected homoserine (Hse) is converted to γ-chloro-homoalanine (γCl-hAla) [18] , was performed in a mixture of PPh 3 and CCl 3 CN in dichloromethane (DCM) overnight. Surprisingly, chlorination treatment also removed the p -methylbenzyl (MeBzl) protecting group of the Sec residue in precursor 2 , thus yielding diselenide 5 upon trifluoroacetic acid (TFA) cleavage. Likewise, the chlorinated intermediate 6 was prepared from Cys-peptide 3 , while on-resin bromination of precursor 4 with PPh 3 Br 2 transformed the TBDMS-protected Hse to a γ-bromo-homoalanine to give 7 in moderate yield. A similar bromination step was unsuccessful for peptides 2 and 3 . Using Boc chemistry, the resin-bound 8 containing bromide and Sec moieties was prepared by coupling of Fmoc-γBr-hAla [21] 9 during peptide assembly as illustrated in Fig. 2b . Removal of the N -terminal Fmoc group using piperidine and subsequent cleavage from the resin by HF acidolysis afforded precursor 10 in modest yield. In a more efficient synthesis, the chlorinated Se-precursor 11 was prepared by Boc chemistry utilizing the β-chloro-alanine and selenohomocysteine (SeHcy, hU)-building blocks during peptide assembly ( Fig. 2c ). 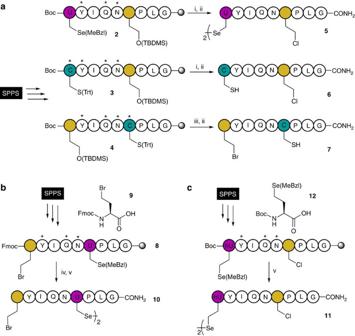Figure 2: Synthesis of the linear halogenated Sec- and Cys-containing OT precursors. (a) By Fmoc chemistry via chlorination or bromination on resin. (b) By Boc chemistry with coupling of a Fmoc-γBr-hAla residue. (c) By Boc chemistry via coupling of a β-chloro-alanine and SeHcy residues. Asterisks indicate that standard side-chain-protecting groups were used for the respective residues during SPPS. Reagents and conditions: (i) PPh3/CCl3CN, DMF, overnight; (ii) TFA:TIS:H2O, 2 h; (iii) PPh3Br2, DCM, overnight; (iv) 20% piperidine in DMF, 1 min; (v) HF:p-cresol (9:1), 0 °C, 1 h. Figure 2: Synthesis of the linear halogenated Sec- and Cys-containing OT precursors. ( a ) By Fmoc chemistry via chlorination or bromination on resin. ( b ) By Boc chemistry with coupling of a Fmoc-γBr-hAla residue. ( c ) By Boc chemistry via coupling of a β-chloro-alanine and SeHcy residues. Asterisks indicate that standard side-chain-protecting groups were used for the respective residues during SPPS. Reagents and conditions: (i) PPh 3 /CCl 3 CN, DMF, overnight; (ii) TFA:TIS:H 2 O, 2 h; (iii) PPh 3 Br 2 , DCM, overnight; (iv) 20% piperidine in DMF, 1 min; (v) HF: p -cresol (9:1), 0 °C, 1 h. Full size image Selenoether and thioether cyclizations The key feature of the selenoether cyclization step is reduction of the diselenide peptide precursor by dithiothreitol (DTT) with concomitant intramolecular Se -alkylation of the generated selenolate ( Fig. 3a ) [31] . Cyclization of precursor peptides 5 – 7 and 10 – 11 was carried out with 100 μM precursor in sodium phosphate buffer at different pH using 40-fold excess DTT ( Table 1 ). The ring-closing reaction was performed at room temperature (RT) and monitored via analytical reversed phase high-performance liquid chromatography (RP-HPLC). Reduction of the γ-bromo-diselenide precursor 10 gave SeCtt 12 in excellent conversion (80–98% over a wide pH range) ( Fig. 3a,b ). At pH 5–11, 12 was formed within 2 h, whereas several hours were required for reactions at pH 3–4 ( Supplementary Fig. 1 ). In contrast, the reaction time for thiolation using the analogous γ-bromo-thiol-precursor 7 took 2–4 times longer and macrocyclization was diminished (Fig. 3b ). Under optimal conditions, γBr-hAla Cys-intermediate 7 was 42% converted to Ctt 13 (pH 11), while γBr-hAla Sec-precursor 10 was quantitatively converted to SeCtt 12 (98%) at pH 5.5 ( Fig. 3c ). The formation of the selenoether or thioether ring was slower (8–72 h depending on pH) using γCl-hAla in comparison with the bromo-counterpart ( Supplementary Fig. 1 ). The γCl-hAla Sec peptide 5 cyclized to SeCtt 14 in 68–86% transformation, while its cysteine-containing counterpart γCl-hAla Cys-peptide 6 cyclized to Ctt 15 poorly (< 32%) even at basic pH ( Fig. 3b ). SeCtt 12 was also produced from 11 ; however, in this case, the intramolecular S N 2 substitution was only effective under basic conditions due to lower reactivity of the SeHcy synthon ( Fig. 3b ). Nevertheless, selenoether formation proceeded smoothly over 72 h at pH 8.3 with no detectable deterioration of the β-chloro-alanine moiety ( Fig. 3c ). 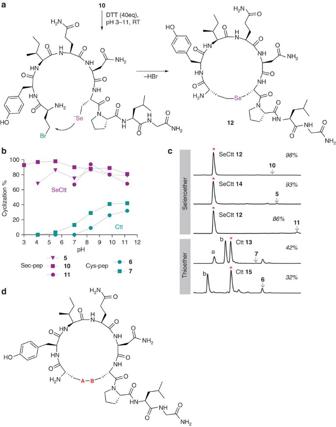Figure 3: Selenoether and thioether cyclizations. (a) Schematic representation of the cyclization of γ-bromo seleno-precursor10to selenoether12. (b) Conversion (%) of the precursors10,5,11,6and7into the respective cyclic products (Table 1) under DTT-reductive conditions at variable pH determined using HPLC. (c) HPLC analysis of the cyclization reaction under optimal conditions (Ctt13and15, pH 11; SeCtt12, pH 5.5 (from precursor10) and pH 8.3 (from precursor11); SeCtt14, pH 5.5). Asterisks mark the retention time for the cyclic products, while arrows indicate retention time of the respective linear precursors. The numbers in italics are the extent of conversion (%) of the linear precursor into the respective macrocycle. Major side products found during thioether cyclization (Fig. 1a) are indicated as peak ‘a’ (fragmentation by intramolecular lactonization) and ‘b’ (hydrolysis to homoserine). (d) General structure of the cyclic OT analogues. A, B: seeTable 1. Figure 3: Selenoether and thioether cyclizations. ( a ) Schematic representation of the cyclization of γ-bromo seleno-precursor 10 to selenoether 12 . ( b ) Conversion (%) of the precursors 10 , 5 , 11 , 6 and 7 into the respective cyclic products ( Table 1 ) under DTT-reductive conditions at variable pH determined using HPLC. ( c ) HPLC analysis of the cyclization reaction under optimal conditions (Ctt 13 and 15 , pH 11; SeCtt 12 , pH 5.5 (from precursor 10 ) and pH 8.3 (from precursor 11 ); SeCtt 14 , pH 5.5). Asterisks mark the retention time for the cyclic products, while arrows indicate retention time of the respective linear precursors. The numbers in italics are the extent of conversion (%) of the linear precursor into the respective macrocycle. Major side products found during thioether cyclization ( Fig. 1a ) are indicated as peak ‘a’ (fragmentation by intramolecular lactonization) and ‘b’ (hydrolysis to homoserine). ( d ) General structure of the cyclic OT analogues. A, B: see Table 1 . Full size image Table 1 Linear precursors to the cyclic OT analogues. Full size table On the basis of the results obtained for synthesis of the linear precursors and their cyclization efficiency, we chose the chloro-peptides 11 and 5 for preparative synthesis of SeCtt OT analogues 12 and 14 , respectively. DTT-induced cyclization was performed directly on crude peptides after cleavage from resin. Selenoether crosslinking of 5 at pH 5.5 gave pure SeCtt 14 in 42% overall yield, whereas precursor 11 at pH 8.3 gave pure SeCtt 12 in 27% overall yield. All compounds were purified to >95% purity via RP-HPLC and characterized using mass spectrometry and nuclear magnetic resonance (NMR). Thermal and plasma stability of the selenoether OT analogues To evaluate their chemical stability, OT peptides were submitted to thermal stress at 55 °C, pH 7.2 ( Fig. 4a ). Native OT degraded significantly over 3 days at 55 °C, with a half-life of 2.2 days, as a result of disulphide bond disruption [32] . These side reactions were not observed with the SeCtt analogues and linkages remained mostly intact under these conditions (calculated half-lives for SeCtts 12 and 14 were 51.3 and 11.3 days, respectively). Metabolic stability studies yielded a half-life of 16 h for OT in human serum at physiological pH and 37 °C ( Fig. 4b ), whereas the half-lives for SeCtt 12 and 14 decay was 60 and 50 h, respectively. The three- to four fold increase in plasma stability is similar to that reported for Ctt 13 (ref. 16 ). 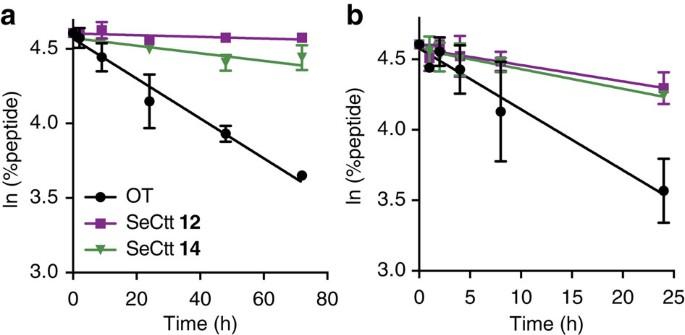Figure 4: Selenoether analogues are more stable than native OT. (a) Thermal stability of OT and SeCtt analogues12and14at pH 7 and 55 °C. (b) Stability of OT and analogues12and14in human plasma. Peptide levels were quantified using LC-MS (n=3). All data are Mean±SEM. Figure 4: Selenoether analogues are more stable than native OT. ( a ) Thermal stability of OT and SeCtt analogues 12 and 14 at pH 7 and 55 °C. ( b ) Stability of OT and analogues 12 and 14 in human plasma. Peptide levels were quantified using LC-MS ( n =3). All data are Mean±SEM. Full size image Functional activity of the selenoether OT analogues The pharmacological activity of native OT, Ctt and SeCtt OT was assessed in a functional Ca 2+ mobilization assay using the human neuroblastoma cell line SH-SY5Y that endogenously expresses OT receptors [33] . All SeCtt and Ctt OT analogues showed similar agonist activity to the parent hormone ( Supplementary Table 1 ). In comparison, the selenoether derivative SeLan 16 , an OT surrogate with a selenolanthionine linker ( Table 1 ) whose synthesis we recently reported [31] , showed loss of bioactivity. NMR structure analysis of OT and selenoether OT 14 and 16 Currently, there are two crystal structures available for OT unbound desamino-OT [34] and a complex of OT with its carrier protein neurophysin [35] . These OT structures are very different; the bound form reveals a helical fold for the OT ring, while the free form is more consistent with β-sheet structure (displaying Type II and III β-turns). The first NMR studies of OT conducted in the 1970s led the authors to propose a flexible structure for OT based solely on temperature coefficients and chemical shift information [36] . Later, NMR studies of OT were focused on its conformation when bound to neurophysin [37] . This latter study reported a lack of inter-residue dipolar connectivities in the absence of neurophysin, and subsequent studies have therefore assumed that OT is flexible and unstructured in solution [38] . This has led to the suggestion that binding to the OT receptor may occur through a receptor-induced fit [34] . Here we re-examined the solution structure of free OT using multidimensional heteronuclear NMR spectroscopy at ultra-high field (900 MHz). The use of ultra-high magnetic field in combination with a cryogenically cooled probe enabled us to overcome the lack of cross peaks observed in nuclear Överhauser enhancement spectroscopy (NOESY) spectra acquired on less sensitive, lower-field instruments [38] . The frequencies of all 1 H atoms (except those absent due to fast exchange with solvent) were assigned using homonuclear total correlation spectroscopy and NOESY spectra, while all protonated heteroatoms were assigned using heteronuclear HSQC spectra. The selenoether bond was assigned using a 1 H- 77 Se HMQC spectrum, where correlations from the Se atom could be observed to protons of neighbouring carbon atoms ( Fig. 5a ) [39] . Structures were calculated using the torsion angle dynamics program CYANA 3.0 (ref. 40 ) using torsion angle restraints derived from 1 H/ 13 C/ 15 N chemical shifts and distance restraints derived from 1 H– 1 H NOEs. The results are summarized in Fig. 5 and Supplementary Tables 2,3 . 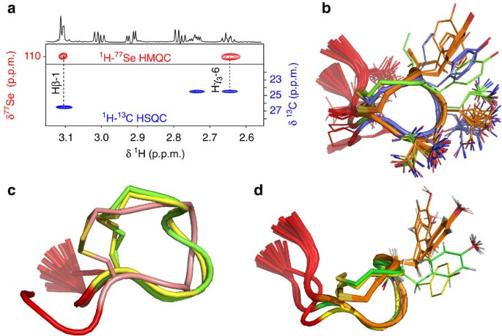Figure 5: Structural characterization. Structural characterization of OT and selenium analogues by NMR at 298 K and comparison to crystal structures. (a) Portions of1H-77Se HMQC and1H–13C HSQC spectra of the bioactive selenoether14. The1H–13C HSQC spectrum shows correlations between the β carbons and their attached protons (at1H frequency of 900 MHz). The1H-77Se HMQC spectrum shows correlations between the Se atom and protons two bonds away (at1H frequency of 500 MHz). A 900-MHz 1D1H NMR spectrum is shown above the 2D spectra. There are clear correlations between the Se atom and β protons on either side of the selenium bridge, confirming its position. (b) Ensemble of 10 NMR-derived solution structures for14(green), the inactive SeLan16(orange) and synthetic OT (blue). The flexible C-terminus is shown in red. (c) Overlay of the OT ring (residues 1–6) of14(green) and the crystal structure of ‘free’ (pink, PDB ID 1XY2) and bound OT (yellow, PDB ID 1NPO). (d) Overlay of the ring (residues 1–6) of active14(green), inactive16(orange) and bound OT (yellow) showing the difference in the position of the Se bridge. Figure 5: Structural characterization. Structural characterization of OT and selenium analogues by NMR at 298 K and comparison to crystal structures. ( a ) Portions of 1 H- 77 Se HMQC and 1 H– 13 C HSQC spectra of the bioactive selenoether 14 . The 1 H– 13 C HSQC spectrum shows correlations between the β carbons and their attached protons (at 1 H frequency of 900 MHz). The 1 H- 77 Se HMQC spectrum shows correlations between the Se atom and protons two bonds away (at 1 H frequency of 500 MHz). A 900-MHz 1D 1 H NMR spectrum is shown above the 2D spectra. There are clear correlations between the Se atom and β protons on either side of the selenium bridge, confirming its position. ( b ) Ensemble of 10 NMR-derived solution structures for 14 (green), the inactive SeLan 16 (orange) and synthetic OT (blue). The flexible C-terminus is shown in red. ( c ) Overlay of the OT ring (residues 1–6) of 14 (green) and the crystal structure of ‘free’ (pink, PDB ID 1XY2) and bound OT (yellow, PDB ID 1NPO). ( d ) Overlay of the ring (residues 1–6) of active 14 (green), inactive 16 (orange) and bound OT (yellow) showing the difference in the position of the Se bridge. Full size image All structures had excellent stereochemistry, although residue G9 is an outlier in the Ramachandran plot and poor side-chain rotamers were occasionally observed for residues Y2 and L8. In all structures, a hydrogen bond was identified between the backbone amide proton of residue X6 and the backbone carbonyl oxygen of Y2. An additional hydrogen bond was found between the backbone amide proton of N5 and the carbonyl oxygen of Y2. The backbone chemical shifts of residues 7–9 are consistent with random coil values and were predicted to be dynamic by Talos+ [41] , in agreement with previous studies (region coloured in red in Fig. 5b ) [38] . The unfavourable NMR properties of sulphur make disulphide bonds largely ‘invisible’ in NMR studies [42] ; in contrast, the SeCtt analogue provided structural constraints through 77 Se couplings to neighbouring methylenes while the additional methylene within the hydrophobic core 14 generated extra distance restraints. Analgesic action of OT and selenoether analogues In order to translate these findings to an intact physiological setting and to determine the mechanism of action of OT-induced analgesia in patients with abdominal pain associated with chronic idiopathic constipation [9] or IBS [10] , we determined the level of OT receptor expression in colonic afferent dorsal root ganglion (DRG) neurons and tested the analgesic properties of native OT and the OT analogues SeCtt 12 and SeCtt 14 on sensory nociceptive afferents innervating the colon. First, we examined expression of the OT receptor in colonic afferent neuronal cell bodies. As only 5% of DRG neurons innervate the colon, we used retrograde nerve tracing from the colon wall to specifically identify afferent neurons in the DRG supplying the colon [43] , [44] , [45] . Laser capture microdissection was then used to isolate the labelled neurons from dissociated DRG cultures, giving a pure colonic afferent neuron population. These studies were performed in healthy mice and in a mouse model of post-inflammatory CVH, which was induced with intra-colonic trinitrobenzene-sulphonic acid (TNBS), as described previously [46] , [47] . The TNBS-treated mice were allowed to recover for 28 days, at which stage inflammation had resolved and chronic colonic afferent mechanical hypersensitivity [46] , [47] and hyperalgesia [48] , [49] were evident. We chose this model as it is being increasingly appreciated that gastrointestinal inflammation can precede IBS symptom development and that low-grade inflammation, mast cell infiltration, and immune dysfunction are evident in different subgroups of IBS patients [43] , [50] , [51] , [52] . Furthermore, chronic visceral mechanical hypersensitivity of colonic afferents is implicated in the development and maintenance of visceral pain in IBS [53] , [54] , [55] . As such these mice are termed CVH mice [46] , [47] . Quantitative RT–PCR analysis and gel electrophoresis showed that the OT receptor expression was below the level of detection in healthy thoracolumbar (TL; T10–L1) colonic DRG neurons ( Fig. 6a,b ). In contrast, OT receptor expression was significantly upregulated in colonic TL DRG neurons from CVH mice ( Fig. 6a,b ). We then determined the effects of native OT and the OT analogues on colonic afferent function [56] . We specifically targeted high-threshold nociceptive afferents in the splanchnic (thoracolumbar) pathway as we have shown that they normally respond to noxious levels of colonic distention/contraction [45] , [46] . These afferents are known to become hypersensitive [46] , [47] and hyper-excitable [57] , [58] in models of chronic visceral pain, which translates to increased signaling of noxious colorectal distention (CRD) within the thoracolumbar spinal cord [59] and enhanced behavioural responses to CRD [48] , [49] . We have also shown that specific functional deficits in these afferents translate to reduced sensory responses to noxious CRD in whole-animal studies [45] . Correspondingly, in the current study we show that with in vitro colonic afferent recordings [43] , [44] , [45] , [46] , [47] , [56] native OT, SeCtt 12 and SeCtt 14 had no effect on colonic nociceptor mechanosensitivity in healthy mice ( Fig. 6c–e and Supplementary Fig. 2 ). However, in recordings from nociceptors from CVH mice we found that native OT, SeCtt 12 and SeCtt 14 all significantly and dose-dependently inhibited the mechanical hypersensitivity observed in CVH colonic nociceptors ( Fig. 6f–h and Supplementary Fig. 2 ). Overall, both SeCtt 12 and SeCtt 14 caused greater inhibition of colonic nociceptors than that induced by native OT ( Fig. 6i–k and Supplementary Figs 2,3 ). Notably, we also found that the inhibitory effect of SeCtt 14 can be blocked by prior luminal administration of the OT receptor antagonist, atosiban ( Supplementary Fig. 4 ). 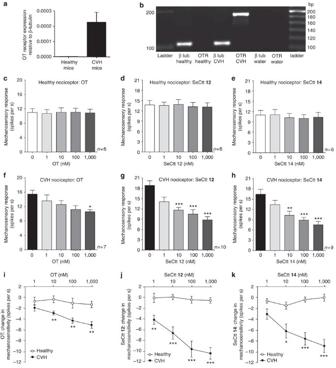Figure 6: OT receptor expression and function in colonic nociceptors during CVH. (a) Colonic DRG neurons from healthy mice lack OT receptor (OTR) expression (below the level of qRT–PCR detection), whereas expression of OT receptors is highly upregulated in colonic DRG neurons from CVH mice. (b) Gel electrophoresis confirming the lack of detectable OT receptor in healthy colonic DRG neurons, but expression in colonic DRG neurons from CVH mice. (c–e)In vitroluminal application of native OT (c), SeCtt12(d) and SeCtt14(e) had no effect at any dose on colonic nociceptor mechanosensitivity in healthy mice (P>0.05). (f) In CVH mice, native OT inhibits nociceptor mechanosensitivity (*P<0.05,n=7). (g,h) In CVH mice, SeCtt12(g) and SeCtt14(h) caused a dose-dependent inhibition of colonic nociceptors, fully reversing the mechanical hypersensitivity of CVH mice (**P<0.01, ***P<0.001, one-way analysis of variance, Bonferronipost hoctest). (i) Native OT caused significantly greater nociceptor inhibition in CVH mice compared with healthy mice relative to baseline responses (**P<0.01). (j) SeCtt12caused significantly greater nociceptor inhibition in CVH mice relative to healthy mice at all doses tested (**P<0.01, ***P<0.001). (k) SeCtt14caused significantly greater nociceptor inhibition in CVH mice relative to healthy mice at 10 nM (*P<0.05, 100 nM (***P<0.001) and 1,000 nM (***P<0.001). All data are Mean±SEM. Figure 6: OT receptor expression and function in colonic nociceptors during CVH. ( a ) Colonic DRG neurons from healthy mice lack OT receptor (OTR) expression (below the level of qRT–PCR detection), whereas expression of OT receptors is highly upregulated in colonic DRG neurons from CVH mice. ( b ) Gel electrophoresis confirming the lack of detectable OT receptor in healthy colonic DRG neurons, but expression in colonic DRG neurons from CVH mice. ( c – e ) In vitro luminal application of native OT ( c ), SeCtt 12 ( d ) and SeCtt 14 ( e ) had no effect at any dose on colonic nociceptor mechanosensitivity in healthy mice ( P >0.05). ( f ) In CVH mice, native OT inhibits nociceptor mechanosensitivity (* P <0.05, n =7). ( g , h ) In CVH mice, SeCtt 12 ( g ) and SeCtt 14 ( h ) caused a dose-dependent inhibition of colonic nociceptors, fully reversing the mechanical hypersensitivity of CVH mice (** P <0.01, *** P <0.001, one-way analysis of variance, Bonferroni post hoc test). ( i ) Native OT caused significantly greater nociceptor inhibition in CVH mice compared with healthy mice relative to baseline responses (** P <0.01). ( j ) SeCtt 12 caused significantly greater nociceptor inhibition in CVH mice relative to healthy mice at all doses tested (** P <0.01, *** P <0.001). ( k ) SeCtt 14 caused significantly greater nociceptor inhibition in CVH mice relative to healthy mice at 10 nM (* P <0.05, 100 nM (*** P <0.001) and 1,000 nM (*** P <0.001). All data are Mean±SEM. Full size image Since native OT and OT analogues SeCtt 12 and SeCtt 14 inhibit colonic nociceptors in vitro , we hypothesized that this inhibition should correspondingly reduce signaling of noxious CRD within the spinal cord in vivo . We administered the OT analogue SeCtt 14 intra-colonically as this route of administration complements the conditions used in our in vitro studies. It also allowed us to ensure peripheral exposure to OT analogue SeCtt 14 for equal time durations, with minimal systemic actions. Furthermore, we recently used this route of administration to demonstrate the preclinical efficacy of a pharmacological treatment that reduces chronic abdominal pain and is poorly systemically absorbed and thus its effects are localized to the gastrointestinal tract [47] . We identified neurons in the dorsal horn (DH) of the thoracolumbar spinal cord activated by noxious CRD ( Fig. 7a and Supplementary Fig. 5 ). In healthy mice, intra-colonic administration of SeCtt 14 had no effect on the number of DH neurons activated in the thoracolumbar spinal cord following noxious CRD ( Fig. 7b–d and Supplementary Fig. 5 ), consistent with the lack of anti-nociceptive effect of native OT and OT analogues we showed in vitro ( Fig. 6 ). In contrast, intra-colonic administration of SeCtt 14 in CVH mice resulted in a significant reduction in the number of DH neurons activated in the thoracolumbar spinal cord following noxious CRD ( Fig. 7e–g and Supplementary Fig. 5 ). Overall, our data indicate that OT analogues reduce nociceptive signaling and reverse chronic visceral mechanical hypersensitivity both in vitro and in vivo but only during states of CVH and not in healthy mice. 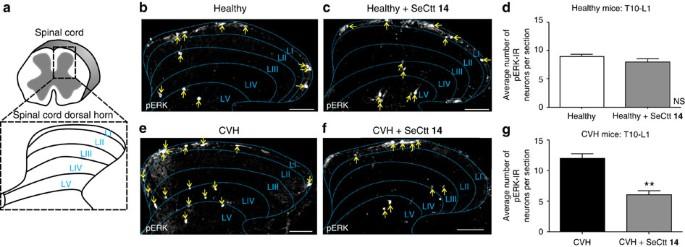Figure 7:In vivostudies. In vivointra-colonic administration of SeCtt14reduces nociceptive signaling, but only during CVH. (a) Schematic representation of laminae I–V (LI–LV) in the dorsal horn of the thoracolumbar spinal cord. (b) In healthy mice, following noxious colorectal distension (CRD), pERK-immunoreactive neurons (pERK-IR; arrows) were predominantly located in laminae I and V of the thoracolumbar spinal cord (T10–L1) (N=6). (c,d) Pretreatment with SeCtt14(1,000 nM) in healthy mice had no significant effect on the number of pERK-IR neurons in thoracolumbar dorsal horn following noxious CRD (N=4). (e) In CVH mice, following noxious CRD (80 mm Hg), more pERK-IR neurons were activated at baseline than in healthy mice and they were predominantly located in the superficial DH laminae I–II and throughout laminae III–V. (f,g) In CVH mice, prior intra-colonic administration of SeCtt14(1,000 nM) significantly reduced the number of pERK-IR DH neurons in dorsal horn of the T10–L1 spinal cord (**P<0.01, CVH:N=6; CVH+SeCtt14:N=4). Group data are combined from 10 sections per T10–T11, T11–T12 and T13–L1 thoracolumbar spinal cord. All scale bars are 100 μm. All data are Mean±SEM. Figure 7: In vivo studies. In vivo intra-colonic administration of SeCtt 14 reduces nociceptive signaling, but only during CVH. ( a ) Schematic representation of laminae I–V (LI–LV) in the dorsal horn of the thoracolumbar spinal cord. ( b ) In healthy mice, following noxious colorectal distension (CRD), pERK-immunoreactive neurons (pERK-IR; arrows) were predominantly located in laminae I and V of the thoracolumbar spinal cord (T10–L1) ( N =6). ( c , d ) Pretreatment with SeCtt 14 (1,000 nM) in healthy mice had no significant effect on the number of pERK-IR neurons in thoracolumbar dorsal horn following noxious CRD ( N =4). ( e ) In CVH mice, following noxious CRD (80 mm Hg), more pERK-IR neurons were activated at baseline than in healthy mice and they were predominantly located in the superficial DH laminae I–II and throughout laminae III–V. ( f , g ) In CVH mice, prior intra-colonic administration of SeCtt 14 (1,000 nM) significantly reduced the number of pERK-IR DH neurons in dorsal horn of the T10–L1 spinal cord (** P <0.01, CVH: N =6; CVH+SeCtt 14 : N =4). Group data are combined from 10 sections per T10–T11, T11–T12 and T13–L1 thoracolumbar spinal cord. All scale bars are 100 μm. All data are Mean±SEM. Full size image In this study, we introduced a methodology for macrocyclization of peptides using non-reducible SeCtt crosslinkers that synthetically overpowers the limited Ctt cyclization strategy. The new procedure utilizes reductant DTT to release the highly reactive selenolate from the diselenide peptide precursor, allowing efficient selenoether crosslinking to take place under mild conditions. The linear peptide precursor can be prepared using either Boc or Fmoc-SPPS with the halogenated moiety incorporated by a chlorination step or coupling of a halogenated building block. Selenide closure is chemoselective and can be applied to unprotected peptides in aqueous media at RT without a catalyst. This approach is particularly promising for the development of disulphide-containing peptide-drug candidates, with the surrogate SeCtt linkage showing substantial higher stability without disturbing the biological active structure of the OT peptide [32] . The structure of ‘free’ OT was determined for the first time by taking advantage of the unprecedented sensitivity of modern NMR spectrometers. Compared with previous studies of OT performed at 600 MHz using a conventional probe, we achieved a fourfold improvement in signal-to-noise by using a cryoprobe-equipped 900-MHz spectrometer (in addition to linear improvements in sensitivity at higher yields). In addition to being able to extract an unprecedented number of dipolar couplings, significant advances in predicting backbone dihedral angles of peptides and proteins based on backbone chemical shifts ( 15 N/ 13 C/ 1 H) allowed us to extract critical backbone φ and ψ angle restraints [41] . The new NMR data revealed that native OT and bioactive SeCtt 12 have similar well-defined structures in aqueous solution; the backbone of the OT rings (residues 1–6) are very similar, whereas the predicted dynamic region overlays poorly (red in Fig. 5 ). Surprisingly, the NMR structures overlay poorly with the crystal structure of the free form of dOT (PDB ID 1XY2) but are in good agreement with the crystal structure of OT bound to its carrier neurophysin. The heterogeneity found in the ‘free’ crystal form has been argued to be due to the inherent conformational flexibility of OT [34] . Furthermore, the large difference between the two crystal forms (0.9 Å) led to the suggestion that OT must undergo a conformational change upon binding its receptor [35] . However, the r.m.s.d. (root mean squared deviation) between the ‘free’ OT crystal structure and the NMR structure is ~1.0 Å, whereas the r.m.s.d. between the NMR structure of the active forms of OT and the complex structure is only 0.3–0.5 Å. This difference is apparent when the backbones of the active OT rings are overlaid: the NMR and neurophysin-bound OT structures overlay well, while the free crystal form is more compressed, perhaps due to crystal packing forces ( Fig. 5c ). Thus, the new NMR data are not consistent with OT undergoing a major conformational change upon binding to neurophysin. Rather, the backbone conformation of OT in aqueous solution appears to be pre-optimized for receptor-binding. However, there are significant differences between the side-chain orientations in the neurophysin-bound OT structure and the NMR structure (0.8–1.1 Å), consistent with these flexible solvent-exposed side chains adopting a thermodynamically more favourable orientation upon binding. The inactive SeLan 16 OT analogue, which has a slightly shorter selenoether bridge in comparison to SeCtt 12 , has a similar overall fold to the other active OT rings, but with small perturbations in the positions of residues 1 and 2. The spatial displacement of the Y2-Cβ atom in SeLan 16 in comparison with the Cβ of bound OT (1NPO) is ~2 Å, while in SeCtt 14 the corresponding displacement is only 0.1 Å. Since the Y2 residue is critical for OT activity, these small structural changes might explain the loss of agonist activity in SeLan 16 . It has generally been assumed that the reported analgesic properties of OT in clinical studies of patients with abdominal diseases [9] , [10] are due to a central effect of OT. However, there is a complete lack of evidence regarding the actual mechanism of action. The work described here reveals a very different scenario, whereby OT and OT analogues can act in the periphery on the endings of nociceptive afferents innervating the colon. In healthy mice, we were unable to detect expression of OT receptors in colonic DRG neurons. However, we found that OT receptor expression is massively upregulated in primary sensory DRG neurons innervating the colon from mice with CVH. Consistent with this high-level expression of OT receptors in CVH, in vitro luminal administration of native OT and the stable SeCtt OT analogues 12 and 14 were anti-nociceptive, as evidenced by their ability to reduce colonic nociceptor mechanosensitivity in a mouse model of chronic abdominal pain ( Fig. 6g,h ). This inhibitory effect was also blocked by the OT receptor antagonist atosiban, which was also applied to the lumen of the colon. This is an important finding as peripheral sensitization of nociceptors has been shown to occur in IBS patients, which contributes to the chronic nature of their symptoms [54] , [55] . This enhanced peripheral signaling facilitates aberrant processing within the spinal cord [59] , which influences the manifestation of pain referred to other organs. Therefore, reducing peripheral signaling is an important component of symptom treatment. Our results represent the first definitive report of native OT, OT analogues and OT receptor actions specifically on peripheral sensory afferent endings in the colon. Critically, our in vitro data show that local luminal absorption of native OT and OT analogues in gut tissue significantly reduces colonic nociceptor function, without the need for systemic effects, but only under conditions of chronic abdominal pain. Correspondingly, we also show that intra-colonic luminal application of OT analogues in vivo significantly reduces signaling from colonic nociceptors into the spinal cord but again only under conditions of chronic abdominal pain. We found that mice intra-colonically administered with the OT analogue SeCtt 14 have a reduced capacity to detect and signal noxious CRD, as indicated by the reduction in activated DH neurons within the thoracolumbar spinal cord. In particular, fewer activated neurons were detected in the superficial lamina of the DH, which is the major termination zone for nociceptive afferents and consists of nociception-specific neurons responding to noxious inputs from afferent fibres [59] . Importantly, the OT analogue SeCtt 14 does not completely inhibit the capacity to signal noxious CRD into the spinal cord in CVH mice; however, it does reduce sensitivity to equivalent healthy levels. This is important, given the physiological importance of these afferents to detect and alert us to harmful events. Since we applied OT analogues to the lumen of the colon over a relatively short time period in both our in vitro and in vivo studies, their actions are predominantly localized in a topical manner to the gut wall. As such, we suggest that native OT and OT analogues act on the peripheral endings of nociceptors innervating the wall of the colon, thereby reducing the nociceptive signal at the first step of the pain pathway. This is an important finding, as targeting peptide therapeutics with poor oral bioavailability to the gastrointestinal tract has been demonstrated to be an effective approach for the clinical treatment of abdominal pain in IBS patients [47] . Such approaches maximize the anti-nociceptive effect of analgesic drugs to the site of action, the peripheral endings of nociceptors in the colon wall, while reducing the risk of systemic side effects. In this study, using the same approach, we identified anti-nociceptive actions of native OT and OT analogues that are of predictive clinical value for the treatment of chronic abdominal pain. Our findings are consistent with previous human studies where OT administration had no effect on pain thresholds in healthy subjects [60] but reduced chronic abdominal pain and discomfort in patients with IBS or chronic idiopathic constipation [9] , [10] . Importantly, the current study provides a mechanistic basis for these contrasting effects, whereby OT receptor expression and function are significantly increased on colonic nociceptors during states of chronic abdominal pain. In conclusion, we improved OT stability by incorporating an isosteric non-reducible selenoether bond and revealed an unprecedented well-defined structure for free OT in solution that might guide future development of mimetics. We demonstrated that OT receptors are massively upregulated in mice with CVH and that the selenoether OT analogues, which are more resistant to redox degradation in the gut environment [61] , [62] than native OT, have analgesic activity in this model of chronic abdominal pain. Peptide synthesis Detailed procedures for the solid-phase assembly, cleavage and purification of the peptides are described in Supplementary Methods . Synthesis of [UYIQN(γCl-hAla)PLG- CONH 2 ] 2 (5) The peptide sequence Boc-Sec(MeBzl)-Tyr(OtBu)-Ile-Gln(Trt)-Asn(Trt)-Hse(OTBDMS)-Pro-Leu-Gly 2 was assembled on a Rink Amide-MBHA resin following the general Fmoc-SPPS procedure ( Supplementary Methods ). Chlorination of the Hse residue was performed as follow: PPh 3 (10 equiv.) and Cl 3 CCN (10 equiv.) were dissolved in DCM (1 ml per 0.1 g resin) at 0 °C. The cold solution was added to the resin and chlorination was carried out overnight at RT. Finally, the peptide was cleaved off the resin and purified using RP-HPLC or used directly for cyclization without further purification. HR-MS calculated for [C 88 H 136 Cl 2 N 24 O 24 Se 2 +2H] 2+ : 1072.4006; found 1072.3978. Synthesis of CYIQN(γCl-hAla)PLG- CONH 2 (6) The peptide sequence Fmoc-Cys(Trt)-Tyr(BrZ)-Ile-Gln(Trt)-Asn(Trt)-Hse(OTBDMS)-Pro-Leu-Gly 3 was assembled on a Rink Amide-MBHA resin following the general Fmoc-SPPS procedure ( Supplementary Methods ). After full assembly of the peptide, the Fmoc group was removed by standard treatment with piperidine. Boc protection of the free N -terminal amine was carried out by treatment of the resin with Boc 2 O (10 equiv.) and N , N -Diisopropylethylamine (DIPEA) (10 equiv.) in N , N -Dimethylformamide (DMF) for 10 min. The Boc group is preferred over the Fmoc group for protecting the N-terminal amino group in order to avoid any future exposure of the generated chloride moiety to base media. Chlorination was carried out by treating the resin with PPh 3 (10 equiv.) and Cl 3 CCN (10 equiv.) in DCM overnight as described for compound 5 . Finally, the peptide was cleaved from the resin and purified using RP-HPLC. HR-MS calculated for [C 44 H 69 ClN 12 O 12 S+H] + : 1025.4640; found 1025.4615. Synthesis of (γBr-hAla)YIQNCPLG- CONH 2 (7) The peptide sequence Fmoc-Hse(OTBDMS)-Tyr(OtBu)-Ile-Gln(Trt)-Asn(Trt)-Cys(Trt)-Pro-Leu-Gly was assembled on a Rink Amide-MBHA resin following the general Fmoc-SPPS procedure ( Supplementary Methods ). After removal of the Fmoc group of Hse1 by standard treatment with piperidine, Boc protection of the free N -terminal amine was carried out by treatment of the resin with Boc 2 O (10 equiv.) and DIPEA (10 equiv.) in DMF for 10 min. Bromination of the Hse residue in 4 was performed by treating the resin with PPh 3 Br 2 (10 equiv.) in DCM (1 ml per 0.1 g resin) at RT overnight. Finally, the peptide was cleaved from the resin and purified using RP-HPLC. HR-MS calculated for [C 44 H 69 BrN 12 O 12 S+H] + : 1071.4115/1069.4135; found 1071.4106/1069.4112. Synthesis of [(γBr-hAla)YIQNUPLG- CONH 2 ] 2 (10) The peptide sequence Tyr(BrZ)-Ile-Gln-Asn-Sec(MeBzl)-Pro-Leu-Gly was assembled on an MBHA resin using Boc-SPPS ( Supplementary Methods ). Upon removal of the Boc group of Tyr2, the resin was treated twice with 5% DIPEA in DMF for 2 min then washed with DMF. Fmoc-γ-bromo-homoalanine 9 21 was coupled by combining the amino acid (5 equiv.) with HOAt (5 equiv.) and DIC (5 equiv.) in DMF:DCM (1:1). The resulting solution was added immediately to resin and the reaction mixture was shaken slowly for 2 h. The solvent was drained and the coupling procedure was repeated. After washing the resin with DMF, the N -terminal Fmoc group was removed by treatment with 20% piperidine in DMF for 1 min (2 × ). TFA cleavage of resin afforded crude peptide that was purified using RP-HPLC. HR-MS calculated for [C 88 H 136 Br 2 N 24 O 24 Se 2 +2H] 2+ : 1116.3501/1117.3481; found 1116.3483/1117.3455. Synthesis of [(hU)YIQN(βCl-Ala)PLG- CONH 2 ] 2 (11) The peptide sequence Boc-SeHcy(MeBzl)-Tyr(BrZ)-Ile-Gln-Asn-[βCl-Ala]-Pro-Leu-Gly was assembled on an MBHA resin using Boc-SPPS ( Supplementary Methods ). The β-chloro-alanine residue at position 6 was coupled in the following way: after removal of the Boc group in Pro3, the resin was treated twice with 5% DIPEA in DMF for 2 min and then washed with DMF. Boc-β-chloro-alanine (5 equiv.) was preactivated for 2 min with HOAt (5 equiv.) and DIC (5 equiv.) in DMF:DCM (1:1) and then coupled to the resin for 1 h. Upon complete assembly of the nonapeptide, HF cleavage of the resin afforded the crude peptide, which was either purified using RP-HPLC or used directly for cyclization without further purification. HR-MS calculated for [C 88 H 136 Cl 2 N 24 O 24 Se 2 +2H] 2+ : 1072.4006; found 1072.3985. Cyclization of the peptides under various pH conditions Linear peptides ( 5 , 6 , 7 , 10 or 11 ) were dissolved in 0.1% TFA solution to a concentration of 1 mg ml −1 . The peptide solutions were then diluted 10-fold in a buffer solution containing DTT (40 equiv. for selenoether cyclization; 20 equiv. for thioether cyclization). The buffer solutions used were as follows: 0.1 M sodium phosphate buffer pH 3.0, 4.1, 5.5, 7.0, 8.3 or 9.8 or aqueous Na 2 CO 3 (5 mg ml −1 , pH 11.2). Cyclizations were carried out at RT and monitored using RP-HPLC. Areas of peaks in analytical HPLC chromatograms were measured and used to quantify the ratio of starting material, cyclized product and side products and to determine the percentage conversion of linear precursors into cyclic products. Supplementary Figure 1 shows the reaction time for the seleno-peptides at different pH. It was important to check the level of DTT consumption throughout the cyclization step. Extra DTT (40 equiv.) was occasionally added to the reaction whenever total conversion of this reagent to its oxidized form was detected using RP-HPLC. The presence of DTT during thioether cyclization was not essential for reactions taking less than 6 h to complete; however, it was beneficial for those with longer reaction times. Synthesis of selenoether OT SeCtt (12) Crude peptide 11 (20 mg, 0.00934, mmol) was dissolved in 0.1M sodium phosphate buffer pH 8.3 (200 ml) containing DTT (170 mg). Cyclization was allowed to take place over 3 days at RT, with occasional addition of DTT (170 mg) after the 1-day reaction. The solution was then diluted twofold with water and the final cyclized peptide was purified using RP-HPLC, affording 5.2 mg of SeCtt 12 in 27% overall yield (from first amino acid loading on resin). HR-MS calculated for [C 44 H 68 N 12 O 12 Se+H] + : 1037.4318; found 1037.4295. Synthesis of selenoether OT SeCtt (14) Crude peptide 5 (6.0 mg, 0.0028, mmol) was dissolved in 0.1 M sodium phosphate buffer pH 5.5 (40 ml) containing DTT (50 mg, 0.336 mmol). Cyclization was allowed to take place over 24 h at RT. The solution was then diluted twofold with water and the final cyclized peptide was purified using RP-HPLC, affording 2.45 mg of SeCtt 14 in 42% overall yield (from first amino acid loading on resin). HR-MS calculated for [C 44 H 68 N 12 O 12 Se+H] + : 1037.4318; found 1037.4302. Synthesis of thioether OT Ctt (13) Crude peptide 7 (7.8 mg, 0.0073, mmol) was dissolved in 0.1 M sodium phosphate buffer pH 9.8 (50 ml). Cyclization was allowed to take place over 4 h at RT. The solution was then diluted twofold with water and the final cyclized peptide 13 was purified using RP-HPLC, affording 1.0 mg of 13 (overall yield: 14% from first amino acid loading on resin). HR-MS calculated for [C 44 H 68 N 12 O 12 S+H] + : 989.4873; found 989.4851. Synthesis of thioether OT Ctt (15) Crude peptide 6 (4.1 mg, 0.0040, mmol) was dissolved in a solution of Na 2 CO 3 (5 mg ml −1 , pH 11.2, 30 ml). DTT (12 mg, 0.078 mmol) was added and cyclization was allowed to take place over 3 days at RT. The solution was then diluted twofold with water and the final cyclized peptide was purified using RP-HPLC, affording 0.77 mg of 15 (overall yield: 19% from first amino acid loading on resin). HR-MS calculated for [C 44 H 68 N 12 O 12 S+H] + : 989.4873; found 989.4869. Thermal stability assay OT and SeCtt 12 and 14 were dissolved in 50 mM sodium phosphate buffer pH 7.0 to a concentration of 20 μM. An aliquot (750 μl) of this solution was placed inside a glass vial, sealed and placed in an incubator at 55 °C. Samples (75 μl) were taken at t =0, 2, 9, 24, 48 and 72 h, quenched with 5% TFA solution (20 μl) and analysed using RP-HPLC. The area of the peak corresponding to the starting peptide was measured and plotted as a percentage of the area at t =0 ( Fig. 4a ). The data were plotted as ln (% of remaining peptide) versus time and the pseudo-first-order rate constant for degradation was used to calculate the half-life of the peptides (OT: 52 h, SeCtt 12 : 1,232 h, SeCtt 14 : 272 h). Stability in human plasma Human plasma (Sigma) was centrifuged at 13,000 r.p.m. for 15 min to separate lipids and then pre-warmed to 37 °C for 15 min before use. A 50 μl aliquot of peptide solution (~500 μM in water) was mixed with 300 μl plasma and incubated at 37 °C. Samples (50 μl) were taken at t =0, 1, 2, 4, 8 and 24 h, quenched with 100 μl of 2% TFA/50% acetonitrile in water, cooled at 4 °C for 30 min and then centrifuged at 13,000 r.p.m. for 5 min. The supernatant was analysed via LC-MS using a Thermo Hypersil GOLD C18 2.1 × 100 mm column running at 0.3 ml min −1 with a gradient of 5–50% B over 30 min. Eluting peptides were detected using an API 150 mass spectrometer in positive ion mode within the mass range 400–1,800 Da. The area of the peak corresponding to the starting peptide was measured and plotted as a percentage of the area at t =0 ( Fig. 4b ). The data were plotted as ln (% of remaining peptide) versus time, and the pseudo-first-order rate constant for degradation was used to calculate the half-life of the peptides (OT: 16 h, SeCtt 12 : 60 h, SeCtt 14 : 50 h). Functional activity of the OT analogues Intracellular Ca 2+ mobilization in response to OT and its SeCtt and Ctt analogues was assessed in SH-SY5Y human neuroblastoma cells endogenously expressing OT receptors as previously described [63] . SH-SY5Y cells were routinely cultured in RPMI media supplemented with 15% fetal bovine serum and plated at a density of 50,000 cells per well on black-walled 384-well imaging plates 48 h prior to the assay. After removal of culture media, SH-SY5Y cells were loaded with Calcium 4 No-Wash dye (Molecular Devices, Sunnyvale, CA, USA) diluted in physiological salt solution (composition: NaCl 140 mM, glucose 11.5 mM, KCl 5.9 mM, MgCl 2 1.4 mM, NaH 2 PO 4 1.2 mM, NaHCO 3 5 mM, CaCl 2 1.8 mM, HEPES 10 mM) for 30 min at 37 °C. Ca 2+ mobilization in response to the addition of OT and its selenocysteine analogues was measured using a FLIPR TETRA plate reader (Molecular Devices; excitation/emission: 470–495 nm/515–575 nm) for 300 s. Raw fluorescence values after addition of compounds were converted to ΔF/F values and the maximum increase in fluorescence after addition of compound plotted as a function of concentration using GraphPad Prism (version 5.03, San Diego, CA, USA). To establish concentration-response curves, a 4-parameter Hill equation with variable Hill coefficient was fitted to the data. NMR spectroscopy 1D 1 H NMR spectra and 2D 1 H– 1 H total correlation spectroscopy (mixing time=80 ms), 2D 1 H– 1 H NOESY (mixing time=350 ms) and 1 H– 13 C HSQC NMR spectra were recorded using samples dissolved in 95% H 2 O/5% D 2 O on a Bruker AVANCE spectrometer equipped with a cryogenically cooled probe, operating at 298 K and a 1 H frequency of 900 MHz. All 77 Se experiments were performed at a 1 H frequency of 500 MHz on a Bruker AVANCE system equipped with a broadband probe. The chemical shifts of 77 Se sites were measured using 1 H- 77 Se HMQC spectra; the optimal value of 1 J (77Se-1H) was determined to be 25 Hz. These 2D experiments required, on average, 10 h of data acquistion time. Chemical shifts were referenced to Sec, as previously described [39] . All nonlabile 1 H as well as aliphatic 13 C and 77 Se chemical shifts were assigned ( Supplementary Table 2 ). Structure determination NOESY spectra were assigned and structures were calculated automatically using the torsion angle dynamics program CYANA v3.0 (ref. 40 ). 1 H– 1 H distance restraints from NOESY data were supplemented with φ and ψ dihedral-angle restraints derived from 1 H, 13 C and 15 N chemical shift data (where available) using the program TALOS+ [41] . Three new templates were added to the CYANA default library in addition to a previously derived template for oxidized SEC [39] . The new templates were as follows: (1) a C -terminal amidation template; (2) a template based on selenomethionine where the S-C bond was substituted with Se-C bond properties and the Se atom was deprotonated (SME); (3) a template was generated based on the cysteine template where the S atom was removed (NSC). Thus, the OT analogues were created by fusing the NSC residue with either SEC or SME using distance restraints. Colonic studies For detailed descriptions of the methodology used, see the Supplementary Methods section. Experiments involving animals were approved by the Animal Ethics Committees of the Institute of Veterinary and Medical Science/SA Pathology and The University of Adelaide. CVH model Intra-colonic TNBS (130 μl ml −1 in 30% ethanol, 0.1 ml bolus) was administered as described previously [46] , [47] , [59] . TNBS-treated mice were allowed to recover for 28 days, at which stage inflammation had resolved and chronic colonic afferent mechanical hypersensitivity was evident. These mice are termed CVH mice. For more information, see the Supplementary Methods . In vitro colonic primary afferent recording preparation In vitro single-unit extracellular recordings of action potential discharge were made from splanchnic colonic afferents. These recordings were made from C57BL/6 healthy or CVH mice using standard protocols [43] , [44] , [45] , [46] , [47] , [56] . Baseline mechanosensitivity was determined in response to application of a 2-g von Frey hair (vfh) probe to the afferent receptive field for 3 s. This process was repeated three to four times, separated each time by 10 s. Mechanosensitivity was then re-tested after the application of native OT (1, 10, 100 or 1,000 nM) or the OT analogues SeCtt 12 (1, 10, 100 or 1,000 nM) or SeCtt 14 (1, 10, 100 or 1,000 nM), respectively. In all cases, peptides were applied to the mucosal surface of the colon for a period of 5 min at each concentration via a small metal ring placed over the receptive field of interest. In some experiments, the OT receptor antagonist atosiban (10 μM) was pre-incubated on the colonic lumen for 10 min before the addition of a combination of atosiban (10 μM) and SeCtt 14 (100 nM). Data are presented as spikes per s and are expressed as mean±s.e.m. n indicates the number of individual afferents. Retrograde labelling to identify colonic neurons in DRG Healthy and CVH mice of 16 weeks of age were anaesthetised with halothane and following midline laparotomy, three injections (10 μl total, 26 s gauge Hamilton syringe) of the fluorescent retrograde neuronal tracer cholera toxin subunit B conjugated to AlexaFluor-555 (CTB AF-555; Invitrogen, Carlsbad, CA, USA; 0.5% in 0.1 M phosphate buffer saline (PBS), pH 7.4) were made sub-serosally within the wall of the descending colon ~2 cm from the anus [44] , [45] , [59] . The viscera were carefully rinsed with sterile saline after each injection to ensure that dye was not incorporated into structures other than the colon wall, and the overlying muscle and skin were then sutured closed. Following surgery, but prior to regaining consciousness, mice were given an analgesic (5 mg kg −1 butorphanol subcutaneously; Intervet, Australia) and an antibacterial (10 mg kg −1 oxytetracycline; Pfizer, Groton, CT). Dissociated DRG cell culture, laser capture microdissection Mice were killed by CO 2 inhalation and DRGs from T10–L1 were surgically removed 4 days after injections of fluorescent dye into the colon (CTB-AF-555). DRGs were digested with 4 mg ml −1 collagenase II (GIBCO, Invitrogen) and 4 mg ml −1 dispase (GIBCO) for 30 min at 37 °C, followed by 4 mg ml −1 collagenase II for 10 min at 37 °C [44] , [45] . Neurons were mechanically dissociated into a single-cell suspension via trituration through fire-polished Pasteur pipettes. Neurons were re-suspended in Hanks’ buffered salt solution (GIBCO) and spot-plated on 50-mm Zeiss duplex dishes (Carl Zeiss, Oberkochen, Germany) and then maintained at 37 °C in 5% CO 2 for 2 h, allowing optimal cell adhesion [44] , [45] . Retrogradely labelled neurons were isolated using a PALM Microlaser Technologies microdissection system (Carl Zeiss) and catapulted directly into a lysis/stabilization buffer-containing carrier RNA (4 ng l −1 ) (Qiagen, Valencia, CA, USA). RNA was isolated from LCM cells using an RNeasy Micro-Kit (Qiagen) following the manufacturer’s instructions. Quantitative RT–PCR Quantitative reverse transcription–polymerase chain reaction (qRT–PCR) was performed using a Chromo4 (MJ Research, Waltham, MA) real-time instrument attached to a PTC-200 Peltier thermal cycler (MJ Research) and Opticon Monitor software (MJ Research). Qiagen QuantiTect SYBR Green RT-PCR 1-step kits were used according to the manufacturer’s specifications with the primers listed in the Supplementary Methods . Colorectal distention and pERK immunohistochemistry Mice received an enema of either saline or SeCtt 14 (1,000 nM). Ten minutes later, under anaesthesia, a 4 cm CRD balloon catheter was inserted transanally into healthy or CVH mice. After regaining consciousness, CRD was performed (80 mm Hg for 10 s, then deflated for 5 s and repeated five times). Following killing via anaesthetic overdose, mice underwent fixation by transcardial perfusion, and the thoracolumbar (T10–L1) spinal cord was removed and cryoprotected. Frozen sections were cut and incubated with monoclonal rabbit anti-pERK with AlexaFluorR488 used for visualization. How to cite this article: de Araujo, A. D. et al. Selenoether oxytocin analogues have analgesic properties in a mouse model of chronic abdominal pain. Nat. Commun. 5:3165 doi: 10.1038/ncomms4165 (2014).